Role of PDGFRA+cells and a CD55+PDGFRALofraction in the gastric mesenchymal niche PDGFRA-expressing mesenchyme supports intestinal stem cells. Stomach epithelia have related niche dependencies, but their enabling mesenchymal cell populations are unknown, in part because previous studies pooled the gastric antrum and corpus. Our high-resolution imaging, transcriptional profiling, and organoid assays identify regional subpopulations and supportive capacities of purified mouse corpus and antral PDGFRA + cells. Sub-epithelial PDGFRA Hi myofibroblasts are principal sources of BMP ligands and two molecularly distinct pools distribute asymmetrically along antral glands but together fail to support epithelial growth in vitro. In contrast, PDGFRA Lo CD55 + cells strategically positioned beneath gastric glands promote epithelial expansion in the absence of other cells or factors. This population encompasses a small fraction expressing the BMP antagonist Grem1 . Although Grem1 + cell ablation in vivo impairs intestinal stem cells, gastric stem cells are spared, implying that CD55 + cell activity in epithelial self-renewal derives from other subpopulations. Our findings shed light on spatial, molecular, and functional organization of gastric mesenchyme and the spectrum of signaling sources for epithelial support. Long-lived gastric and intestinal stem cells produce distinct differentiated cell types within stereotypic monoclonal crypts (intestine) or glands (stomach). Lgr5 -expressing intestinal stem cells (ISCs) at the base of each crypt drive brisk cell turnover [1] , [2] . The epithelium of the gastric antrum, the region nearest the intestine, lacks villi but turns over almost as rapidly as intestinal epithelium; each gland consists mainly of mucus-producing foveolar cells that line luminal “pits” and distinct mucous cells at the base. Like ISCs, antral epithelial stem cells lie near the gland base (Fig. 1a ), express Lgr5 , and replicate symmetrically [3] , [4] , [5] , [6] ; it is, however, unclear whether Lgr5 marks dedicated multipotent cells or basal mucous cells with facultative stem-cell properties [7] ; other candidate stem cell genes, such as Vil1 , Runx1 , Sox2 , Axin2 and Aqp5 , express in partially overlapping compartments [4] , [7] , [8] , [9] , [10] and may also mark facultative or fractions of active stem cells. Diverse observations nevertheless support the view that multipotent antral stem cells reside near gland bottoms and that their progeny mainly migrate upward to replenish the physiologic attrition of terminal foveolar cells (Fig. 1a ) [3] , [4] . Fig. 1: Structure and organization of gastric corpus and antral mesenchyme. a Stomach and intestinal regions and different organizations of glandular stomach epithelia. b Cross-sections of corpus (top) and antrum (bottom), showing smooth muscle actin (SMA1, yellow)-expressing smooth muscle fibers and CD31 + (red) capillaries packed tightly in the stroma between glands (nuclei stained with DAPI, blue). Dashed lines delineate gland lumen. Scale bars 50 μm. Representative images from three independent experiments. c Whole-mount 3D rendering of corpus (left) and antral (right) glands, highlighting structural differences in muscle fibers (SMA1, yellow) and capillaries (CD31, red) in the two regions. Tissue cross-sections at the level marked by dashed lines are shown in the bottom right (DAPI in blue, CD31 in red). Scale bars 50 μm. d Whole-mount 3D rendering of corpus (left) and antral (top right) glands in Pdgfra H2BeGFP mice. Laminin (yellow) marks the basal lamina and highlights gland pits. Tissue cross-sections at the levels marked 1 and 2 are shown in the bottom right, with PDGFRA Hi cells in neon green and PDGFRA Lo cells in light green. Double-headed arrow highlights PDGFRA Lo layer beneath corpus gland bottoms. Immunostaining with PDGFRA antibody (red) shows the extent of PDGFRA + cytoplasm enveloping each gland. Scale bars 50 μm. e Single frames extracted from 3D video renderings of Pdgfra Cre(ER-T2) ;Rosa26 mT/mG mouse (stained green after tamoxifen treatment) corpus (left) and antrum (right) to show the morphology of Pdgfra Hi cells enveloping each gland and additional Pdgfra Lo cells occupying space beneath glands (white arrowheads). Full videos of corpus and antral gland 3D renderings are included in the Supplementary information, see Supplementary Movies 5 and 6 . f Schematic representation of the distributions of PDGFRA Hi (dark green) and PDGFRA Lo (light green) cells in relation to corpus and antral glands. Full size image The corpus epithelium, which turns over slower than antral or intestinal epithelia, also contains surface foveolar cells; the neck of each gland carries mucous neck and acid-secreting parietal cells, while the gland base houses zymogenic “chief” cells (molecular markers we use to identify cell types in this study are listed in Supplementary Fig. 1a ). The isthmus of corpus glands, populated by presumptive stem cells and their transit-amplifying daughters, lies between the pit and the neck (Fig. 1a ); progeny of these replicating cells migrate bidirectionally, pit-cell precursors toward the lumen and other precursors toward the gland base [11] , [12] , [13] . Corpus isthmus stem cells replicate frequently and replenish, at a minimum, the pit and upper neck regions [14] , [15] . A distinct population with stem-cell properties resides among chief cells at the gland base, expresses Wnt pathway genes Troy and Lgr5 , and rarely replicates at rest but becomes activated upon injury to replenish cell losses in the basal and lower neck regions [16] , [17] , [18] , [19] , [20] , [21] . The balance that active and facultative gastric stem cells strike between self-renewal and differentiation reflects the epithelial response to signals from underlying mesenchyme. Active antral stem cells, for example, require Wnt signaling to maintain their state and proliferate [3] , [7] , [22] , and facultative corpus stem cells are recruited to replicate in part by Wnt signaling [16] , [17] . Conversely, bone morphogenetic protein (BMP) signaling drives epithelial differentiation [23] , [24] , [25] and inhibitors of the pathway (BMPi) are implicated in gastric metaplasia and Helicobacter pylori infection [26] , [27] . Whereas recent studies have defined anatomic and functional relations between intestinal stromal and epithelial compartments in increasing detail [28] , [29] , [30] , [31] , [32] , [33] , [34] , [35] , [36] , gastric mesenchyme is as yet superficially characterized. By combining corpus and antral cells, a recent single-cell analysis obscured possible differences between regionally distinct populations [37] . Here we report on our structural, molecular, and functional characterization of whole tissues and single cells from adult mouse corpus and antral mesenchyme. We define notable similarities and differences between epithelial and underlying stromal elements in the corpus, antrum, and small intestine (SI). Focusing on cells that express PDGFRA, we identify sub-glandular CD55-expressing fibroblasts as functional counterparts of intestinal trophocytes in the stomach. Anatomic definition and signaling potential of antrum and corpus mesenchyme Foveolar cells are present in both gastric regions; their fraction is larger in the antrum, where pits (foveolae, outlined by staining with the lectin UEAI or with laminin antibodies) are wider and deeper in relation to the whole gland than those in the corpus (Supplementary Fig. 1b, c ). In both regions, whole-mount confocal imaging revealed blood vessels and smooth muscle fibers packed tightly in the limited space between individual glands (Fig. 1b ). Corpus arterioles branch along the full gland length to extend a deep capillary network, while antral arterioles have a larger bore and extend capillaries mainly at gland tops, with little branching along the gland length (Fig. 1c and Supplementary Fig. 1d, e , Supplementary Movies 1 and 2 ). Slender smooth muscle fibers extend lateral branches near the foveolar base, so the resulting fine network of lamina propria myocytes is taller and wider in the antrum (Fig. 1c and Supplementary Movies 3 and 4 ). Pdgfra -expressing mesenchymal cells are pivotal in intestinal epithelial homeostasis [33] . In Pdgfra H2BeGFP knock-in mice [38] , [39] , we detected cells with high and low levels of nuclear GFP (Fig. 1d and Supplementary Fig. 1e–g ). Antral PDGFRA Hi cells aggregate around the pit, where they extend beyond the basement membrane into the lamina propria (Supplementary Fig. 1e, f ), while corpus PDGFRA Hi cells distribute uniformly along corpus glands (Supplementary Fig. 1g ). PDGFRA Lo cells distribute uniformly along the antral gland length but their density is modestly lower near the corpus isthmus and neck; in both gastric regions, PDGFRA Lo cells also concentrate below the gland base, occupying a substantially larger space in the corpus than in the antrum (Fig. 1d and Supplementary Fig. 1g ). To further assess cell morphology, we crossed Rosa26 mT/mG reporter [40] and Pdgfra Cre(ER-T2) knock-in mice [41] , thus producing mice where baseline red fluorescence (Tomato) in all cell membranes turns green (GFP) in cells with Cre enzyme activity (Supplementary Fig. 2a ). Tamoxifen did not induce structural changes that indicate tissue toxicity (Supplementary Fig. 2a ). Cells embedded in the basal lamina, corresponding to PDGFRA Hi , engulf glands within their intercalated cytoplasmic projections and cells corresponding to PDGFRA Lo are present beneath glands (Fig. 1e and Supplementary Movies 5 and 6 ). In summary, PDGFRA + cells are present throughout the glandular stomach and their different arrangements in the corpus and antrum (Fig. 1f ) likely reflect distinct influences on overlying gastric epithelia. SI crypts form organoid structures in Matrigel supplemented with EGF, Noggin (a BMPi), and RSPO1, a Wnt potentiating agent (ENR medium) [42] . As Lgr5 + stem cells in the antral gland base resemble those in SI crypt bottoms, the original conditions to culture antral glands were adapted from an SI foundation and include additional requirements for Wnt3a and gastrin (ENRWG) [3] . Selected intestinal PDGFRA Lo cells, which express BMP inhibitor (BMPi) and RSPO genes, induce intestinal crypts to form spheroids in vitro in the absence of any supplemental factors [33] . PDGFRA Lo cells isolated by flow cytometry from either gastric segment (Supplementary Fig. 3a ) failed to expand intestinal crypts in vitro, revealing a functional distinction from their intestinal counterparts (Fig. 2a ). In contrast, corpus and antral glands readily formed spheroid structures in the absence of recombinant (r) factors when co-cultured with PDGFRA Lo cells isolated from the SI or from the corresponding gastric region (Fig. 2b ) but not when co-cultured with gastric stromal PDGFRA neg or CD31 + endothelial cells (Supplementary Fig. 3b ). Spheroids arising from corpus glands were consistently smaller and fewer than those from antral glands but expressed corpus-specific (chief and parietal cell) markers, while antral spheroids expressed higher levels of Wnt target genes Axin2 and Cd44 (Supplementary Fig. 3c ). These structures thus reflect region-specific cell differentiation, different degrees of corpus and antral progenitor cell expansion, and discernible effects from mesenchymal cell co-cultures. Because isolated gastric PDGFRA neg cells showed negligible activity in the assay, we focused on characterizing PDGFRA + cells further. Fig. 2: Molecular distinction of corpus and antral PDGFRA-expressing mesenchyme. a Co-culture of SI crypts with PDGFRA Lo cells isolated from SI, antral or corpus mesenchyme and without NOG or RSPO1 (−GF). Stomach PDGFRA Lo cells did not induce spheroids. SI organoid growth in complete ENR served as a control. Scale bars 400 μm. Bars represent mean ± SEM. ENR: n = 9, +SI n = 14, +Corp and +Ant: n = 4. Significance of differences determined by one-way ANOVA and Tukey’s multiple comparison test. ns not significant. Source data provided as a Source Data file. b Co-culture of corpus or antral glands with PDGFRA Lo cells isolated from the same segment or from SI elicited spheroid growth in the absence of rNOG and RSPO1. Scale bars 400 μm. Corpus: ENRWG n = 15, +Corp Lo n = 12, +SI Lo n = 11, Antrum: ENRWG n = 14, +Ant Lo n = 12, +SI Lo n = 13. Control: gastric spheroid growth in ENRWG medium. Bars represent mean ± SEM. Significance of differences determined by one-way ANOVA and Sidak’s multiple comparison test. ns not significant. Source data provided as a Source Data file. c Pearson correlations among RNA-seq libraries from SI, antral, and corpus PDGFRA Hi and PDGFRA Lo cells isolated from Pdgfra H2BeGFP mice. Differences between gastric and intestinal PDGFRA + cells are detailed in Supplementary Data 1 . d Genes differentially expressed ( q < 0.05; log 2 fold-difference >1.5) between SI, antral, and corpus PDGFRA Hi cells. Selected genes are named. Significance of differences determined by DESeq2 default settings (Wald test). e Genes enriched in each regional population ( q < 0.05; log 2 fold-difference >1.5; k -means = 6) and Integrative Genome Viewer tracks for representative genes enriched in antral PDGFRA + cells. Actb controls for normalization of read counts. Parentheses: range of signal values. f Genes differentially expressed ( q < 0.05; log 2 fold-difference >1.5) between antral and corpus PDGFRA Hi and PDGFRA Lo cells. Significance of differences determined by DESeq2 default settings (Wald test). g Relative expression of mRNAs for candidate niche factors (BMP, Wnt, FGF, and EGF agonists and antagonists) in each mesenchymal cell population. Heatmap is prepared from normalized rlog counts from DEseq2; each row represents one replicate. h Bulk RNA-seq data point to a higher BMP tone from Pdgfra + cells in stomach than in the SI. Full size image Regionality of gastrointestinal Pdgfra-expressing mesenchymal cells To define regional differences, first we profiled bulk transcriptomes of PDGFRA + cells purified by flow cytometry from the corpus and antrum of Pdgfra H2BeGFP mice. Stripping external muscle before cell isolation excluded PDGFRA Hi neurons nestled therein, so that the remaining PDGFRA Hi cells represent gastric sub-epithelial myofibroblasts (SEMFs). Replicate RNA-seq libraries from each cell isolation were highly concordant (Supplementary Fig. 3d ). In unsupervised hierarchical analysis, gastric PDGFRA + cells were distinct from their previously described intestinal counterparts [33] , followed by differences between PDGFRA Hi and PDGFRA Lo cells in each organ (Fig. 2c ). Corpus and antral PDGFRA Hi cell (SEMF) transcriptomes resembled each other more than they resembled SEMFs from the SI (Fig. 2d , Supplementary Fig. 3e and Supplementary Data 2 ). Exclusive expression of known transcriptional regulators Barx1 and Pitx1 in gastric, and of Nkx2-3 and posterior Hox genes in intestinal, cells support the veracity of additional findings. For example, gastric SEMFs express higher levels of Fgf7 , Fbln1 and Fbln2 , Cd81 , and transcription factor genes Atf3 and Osr1 , whereas intestinal SEMFs express higher levels of Il33 and Il34 , the Wnt inhibitor Wif1 , and transcription factor Irf8 . Differential expression of Acta2 and Myh11 hints that intestinal and antral SEMFs may be more contractile than those in the corpus. Segment- and cell type-specific gene modules were evident in each population (Fig. 2e ). Intestinal PDGFRA Lo cells have the most distinctive transcriptome of any population, with unique expression of Eln , Col8a1 , and Il6 , among other factors, and differing from intestinal SEMFs in expression of >2100 genes ( q < 0.05; |log 2 fold-change| > 1.5), compatible with distinct and opposing functions [33] (Supplementary Fig. 3f ). The corresponding populations in both corpus and antrum are less divergent, differing in expression of ~800 (antrum) to ~1100 (corpus) genes (Fig. 2f ). Gastric PDGFRA Lo cells from either segment are enriched for Cd55 (a marker we investigate later in this study), Lepr and Dll1 (genes that mark specific mesenchymal cells in mouse and human intestinal mesenchyme, respectively) [43] , [44] while gastric SEMFs are enriched for signaling factors such as Fgf9 and Angptl1 , multiple BMP genes, and for transcription factor (TF) gene Sox6 and, in the antrum, Wnt-responsive Lef1 (Fig. 2d, e and Supplementary Data 2 ). Foxl1 , which marks intestinal SEMFs among other cells [31] , [33] , [45] , is expressed in gastric SEMFs and, at a lower level, also in gastric PDGFRA Lo cells. Thus, regional differences in the spatial arrangements of Pdgfra -expressing cells (Fig. 1 ) extend to their gene expression profiles. Among potential sources of the signals that support epithelial expansion in vitro, genes for canonical Wnt2 and for non-canonical ligands Wnt4 , Wnt5a , and Wnt5b are expressed in both PDGFRA + populations in both corpus and antrum; however, Wnt-potentiating factors Rspo1 , Rspo2 , and Rspo3 express at lower levels in gastric than in intestinal PDGFRA Lo cells (Fig. 2g ). Thus, while PDGFRA + cells in every segment produce Wnt ligands, only transcripts in intestinal PDGFRA Lo cells display a potential for significant canonical Wnt signaling. BMP transcripts are enriched not only in intestinal, antral, and corpus PDGFRA Hi cells, but Bmp2 , Bmp5 , and Bmp7 are also prominent in gastric PDGFRA Lo cells (Fig. 2g ). Grem1 , a BMPi abundant in intestinal PDGFRA Lo cells, and other classical BMPi are barely present in bulk populations of gastric PDGFRA Lo cells, which instead express a putative and atypical BMP7 inhibitor, Ctgf [46] , [47] . Based on mRNA levels alone, these findings suggest that overall BMP “tone” may be higher in the stomach than in the SI (Fig. 2h ). In culture, gastric glands generally form spheroid structures (see Fig. 2b and Supplementary Fig. 3b ), distinct from intestinal organoids, in which budding protrusions represent crypts housing progenitor and stem cells [42] . When conditions to culture gastric glands were first defined, human fibroblast growth factor (FGF) 10 induced budding of unclear significance (stomach epithelium lacks crypts) [3] . In this light, the asymmetry of FGF transcripts in PDGFRA + cells is striking. Of the five transcripts expressed in any population, Fgf9 is expressed in SEMFs and Fgf10 in PDGFRA Lo cells from all sites, while Fgf7 is especially high in antral SEMFs. Nrg1 , an EGF-family factor implicated in ISC regeneration after injury [34] and corpus pit cell differentiation [48] , is also uniquely higher in gastric (especially antral) than in intestinal SEMFs and PDGFRA Lo cells (Fig. 2g ). Transcriptional features of antral and corpus mesenchyme Having identified differences in sub-epithelial structure and signaling capacity, we examined cellular heterogeneity by mRNA profiling of whole gastric mesenchyme (manually depleted of external smooth muscle) at single-cell resolution. A total of 34,445 mesenchymal cells (20,624 from corpus and 13,821 from antrum; epithelial contamination was negligible) provided information on at least 900 transcripts each (2700 transcripts for antrum Rep.1, Supplementary Fig. 4a ). Consistent with the structures and cells revealed by fluorescence microscopy, graph-based clustering identified substantial fractions of Cd31 + endothelial cells from corpus, Acta2 hi Myh11 hi myocytes, Acta2 lo Myh11 lo Rgs5 + pericytes, and PDGFRA + cells that lack these markers (Fig. 3a ). Less than 10% of whole isolates were Ptprc + immune cells, smaller than the 45% fraction present in whole SI mesenchyme [33] , only ~1% of cells were glial, and <1% showed signs of ongoing cell replication (Fig. 3a ). Despite structural differences in corpus and antral blood vessels and muscle fibers (Fig. 1 ), transcriptomes of their constituent cells showed few regional differences. Significant cluster distinctions between corpus and antrum mapped exclusively to Pdgfra + cells (Fig. 3b and Supplementary Fig. 4b ), which express more candidate niche factors than other mesenchyme (Supplementary Fig. 4c ). As all other cell types from corpus and antrum resembled each other similar Pdgfra + cell dissimilarities are unlikely to represent a batch effect, as we confirmed additionally with AUGUR analysis [49] (Supplementary Fig. 4d ). These findings justify our preceding attention and subsequent focus on the 5896 antral and 6594 corpus Pdgfra + cells from our scRNA-seq study. Fig. 3: Delineation of corpus and antral PDGFRA + mesenchymal cell populations. a Left: Uniform manifold approximation and projection (UMAP) plot of mRNA profiles from 34,445 single cells isolated from corpus (20,624 cells) and antral (13,821 cells) mesenchyme. Right: Relative expression of known cell-restricted genes in the UMAP cell clusters. Circle diameters represent the cell fraction expressing a gene and shades of purple represent normalized average expression within the population. b MetaNeighbour AUROC (area under the receiver operating characteristic) analysis shows high similarity between corresponding antral and corpus mesenchymal cells of each type other than the PDGFRA Hi and PDGFRA Lo cell populations. c Left: UMAP identification of distinct populations of Pdgfra -expressing cells extracted from scRNA analysis of unfractionated mesenchyme. Right: Relative expression of Pdgfra and Cd34 in the identified Pdgfra -expressing populations and the corresponding SI cells. Blue, corpus; red, antrum; green, SI. The 3 corpus populations are more distinct than the 3 antral populations. d Differential genes expressed among the six PDGFRA + mesenchymal cell types (Wilcoxon Rank Sum test, logfc.treshold = 0.25). The genes are listed in Supplementary Data 2 . e Relative expression of marker genes from the three antral PDGFRA + subpopulations identified by scRNA-seq. Circle sizes represent the percentage of cells expressing a gene, fill colors represent normalized average expression. AntInt shows distinct intermediate patterns. f Expression of niche genes Bmp7 and Nrg1 in each population compared with Pdgfra -expressing SI mesenchymal cells. AntInt expression levels are comparable to those in antral Pdgfra Hi cells (AntHi). Nrg1 expression in corpus and SI is significantly lower than in antral cells. g Grem1 and Rspo3 expression in each population compared with Pdgfra -expressing SI cells. Both genes are restricted to Pdgfra Lo populations and expressed at lower levels in the stomach than in SI. Full size image Graph-based analysis limited to these cells identified 6 clusters: Pdgfra Hi and two related but distinct Pdgfra Lo cell populations from each gastric segment (Fig. 3c and Supplementary Fig. 2b —note that Cd34 marks intestinal Pdgfra Lo but not Pdgfra Hi cells [33] ). Two Pdgfra Lo cell types in the corpus, CorpLo and CorpLo1, were separated on UMAP graphs but, consistent with bulk RNA profiles (Fig. 2e ), antral cells separated less well. UMAP distinguished antral Pdgfra Hi (AntHi) and Pdgfra Lo (AntLo) cells and a substantial (44% of Pdgfra + cells) third pool, AntInt, with intermediate Pdgfra and Cd34 levels and a distinctive RNA profile (Fig. 3c, d ); this profile includes enriched expression of the transcription factor (TF) gene Sox11 , contractile genes Acta2 and Myh11 , and prostaglandin synthase Ptgs2 (Fig. 3e and Supplementary Data 3 ). Some features resemble AntHi (e.g., EGF-family genes Ereg , Areg and Nrg1 , the TGF-ß inhibitor Tgfbi , and Col4a5 ) and others resemble AntLo (e.g., Tgfb2 , Wnt antagonist Sfrp1 , and extracellular matrix factors Spon2 , Col15a1 , Fbln1 and Fbln2 ). Notably, Bmp2/5/7 and non-canonical Wnt4 transcript levels approach those in antral and intestinal SEMFs ( Pdgfra Hi cells), while other signals (e.g., Wnt5a, Fgf7 ) are lower than in SEMFs (Fig. 3e, f and Supplementary Fig. 4c, e ). Because flow cytometry separated PDGFRA Hi and PDGFRA Lo cells from Pdgfra H2BeGFP mouse corpus better than the antrum (Supplementary Fig. 3a ), we infer that AntInt segregates between these two populations in FACS isolation. The above differences, however, mark them as distinct cells and we show below that they differ from AntLo in niche activity. Differences between corpus and antral Pdgfra Lo subpopulations also include expression of known niche factors. Low levels of intestinal niche factors Grem1 and Rspo3 apparent in bulk RNA profiles of stomach PDGFRA Lo cells (Fig. 2g ) are largely limited to the distinct CorpLo1 cluster and AntLo, albeit at levels lower than intestinal Pdgfra Lo cells (Fig. 3g ). CorpLo1 also expresses a different spectrum of extracellular matrix genes (high Has1 , Dpt and Col14a1 —Supplementary Data 3 ) compared to CorpLo, suggesting that these cells may localize in different anatomic domains. Of note, BMP agonist mRNA levels diverge less between Pdgfra Hi and other Pdgfra + cells in the stomach than in the intestine and BMPi express at lower levels (Supplementary Fig. 4f ), affirming ostensibly higher BMP tone in the stomach. MetaNeighbor showed that AntInt most resembles AntLo (Supplementary Fig. 4g ). In summary, we identify distinct gastric PDGFRA + populations from each region and below we address their properties systematically. Molecular and spatial heterogeneity of antral SEMFs We first considered Pdgfra Hi cells (SEMFs), which occupy a specific anatomic compartment and have unique mRNA profiles (Figs. 1 – 3 ). Gastric and intestinal SEMFs differ in high Fgf7 (antrum) and Fgf9 (corpus) expression and in profiles of the TF genes Foxl1 and Gli1 (Fig. 2g and Supplementary Figs. 4c and 5a ). Considered apart from other mesenchymal cells, they divided into one corpus and two antral subpopulations, all of which express canonical BMP ligand genes (Fig. 4a and Supplementary Fig. 5b ). Notably, one antral cluster expresses high Fgf7 and the EGF ligand Nrg1 , while the other is marked by high Bmp3 and Ctgf (candidate non-canonical BMPi) [50] , [51] and low levels of Nrg1 , a profile similar to corpus SEMFs (Fig. 4a, b ); Fgf7 and Bmp3 are largely SEMF-restricted, while the other genes are enriched in SEMFs but also expressed in other PDGFRA + cells (Supplementary Fig. 4c, f ). In situ hybridization localized antral Fgf7 + Nrg1 + SEMFs to the tops of antral glands, adjacent to foveolae, whereas Bmp3 and Ctgf localize primarily in SEMFs that abut the zone of epithelial cell replication in the lower gland (Fig. 4c ). As antral SEMF density is higher at gland tops than at the base (Supplementary Fig. 1e–g ), the proportions of SEMF subpopulations (Fig. 4a ) further support that molecularly distinct antral SEMF subpopulations are spatially segregated. Fig. 4: Identification and functional assessment of distinct gastric SEMF populations. a In isolation, corpus and antral SEMFs are distinct and antral SEMFs divide further into two cell populations. Right: Fgf7 , Nrg1 , Bmp3 , and Ctgf mRNA densities projected on the UMAP plot. b Relative expression of scRNA-seq markers from the three SEMF populations. Circle diameters and fill colors represent the fraction of cells expressing a gene and normalized average expression levels. The two antral SEMF populations differ in expression of Fgf7, Nrg1 , Bmp3 , and other factors; corpus SEMFs resemble the smaller antral Bmp3 + cluster more than the larger population of antral Fgf7 + Nrg1 + cells. c Fluorescence in situ hybridization (RNAscope) on antral tissue sections localizes Fgf7 - and Nrg1 -expressing PDGFRA Hi SEMFs near gland pits and Bmp3 - and Ctgf -expressing cells in the lower half of glands. Images represent fields examined in three independent experiments with each probe. Scale bars 50 μm. Heatmap: average fluorescence signal quantified along 16–25 individual glands ( Ctgf probe quantification is shown in Fig. 6a ). Source data are provided as a Source Data file. Right: schematic representation of antral SEMF distribution. d Co-culture of antral and corpus glands with unfractionated PDGFRA Hi cells, which fail to induce spheroids in the absence of rNOG and RSPO1. Glands cultured in ENRWG medium serve as controls. Scale bars 400 μm. Bars represent mean ± SEM. Antrum: +ENRWG n = 22, +PDGFRA Hi n = 19, No cells n = 22; Corpus: +ENRWG n = 19, +PDGFRA Hi n = 12, No cells n = 18. n : number of culture wells analyzed over six independent experiments. Significance of differences determined by one-way ANOVA coupled with Sidak’s multiple comparison test. **** p < 0.0001, ns not significant. Source data are provided as a Source Data file. e Antral glands exposed to recombinant rFGF7 or rFGF10 in addition to complete ENRWG medium. Budding of spheroid structures increased upon treatment with rFGF7 without affecting spheroid numbers ( n = 8 independent experiments). Bars represent mean ± SEM. Significance of differences determined by one-way ANOVA coupled with Dunnett’s multiple comparison test. ns not significant. Scale bars 400 μm. Source data are provided as a Source Data file. Full size image Because Bmp3 and Ctgf may have BMPi activity [50] , [51] and SEMFs expressing those genes lie near proliferative epithelial cells, we asked if they might support antral gland growth in vitro; to optimize the assay for BMPi activity, we reduced RSPO and Wnt3 concentrations 5-fold. In these conditions, rNOG readily supported antral spheroids, but the same concentration of human rBMP3 or rat rCTGF lacked that activity (Supplementary Fig. 5c ). No surface marker reliably separated Bmp3 + Ctgf + from Fgf7 + Nrg1 + SEMFs. When co-cultured with gastric glands in the absence of any recombinant factor, unfractionated FACS-sorted antral or corpus PDGFRA Hi cells (GFP Hi cells from Pdgfra H2BeGFP mice) did not induce spheroid growth from the corresponding glands, in contrast to the stimulation by ENRWG medium (Fig. 4 d) or by bulk PDGFRA Lo cells (Fig. 2b ). Together, these findings reveal spatial and molecular asymmetry of antral SEMFs that fail to support corpus or antral gland growth in vitro, much as intestinal SEMFs lack discernible support function in organoid assays [33] . To better define SEMF contributions in those assays, we co-cultured gastric glands with SEMFs in complete ENRWG medium, in medium lacking EGF and Noggin, or in medium containing RSPO1 as the only supplement. In the presence of these factor combinations, SEMFs did not reduce the number of resulting spheroids (Supplementary Fig. 5d ). In cultured antral glands, recombinant human FGF10 induces buds, which are presumed to reflect epithelial maturation [3] . Because Fgf7 is abundant in peri-foveolar antral SEMFs, belongs in the same clade as Fgf10 , and their common receptor, Fgfr2 , is expressed in antral epithelium [52] , we considered a function for FGF7 in epithelial differentiation. Addition of murine rFGF7 to ENRWG medium increased budding substantially without affecting organoid numbers (Fig. 4e ). Although constitutive Fgf7 gene disruption has no reported effects on mouse gastric development or function [53] subtle differentiation defects could have been masked. To assess possible gastric functions in adult mice, we used CRISPR gene editing to flank exon 2 of the Fgf7 locus with LoxP sites (Supplementary Fig. 6a ), then introduced the floxed allele onto the Pdgfra Cre(ER-T2) background [41] . Pdgfra Cre(ER-T2) ;Rosa26 LSL-tdTomato mouse stomachs revealed robust Cre recombinase activity in PDGFRA Hi and, at lower efficiency, in PDGFRA Lo cells (Supplementary Fig. 6a , see also Fig. 1e and Supplementary Movies 5 and 6 ). PCR genotyping verified the expected null allele in Tomato + cells isolated from antral Pdgfra Cre(ER-T2) ;Fgf7 Fl/Fl ;Rosa26 LSL-TdTomato mesenchyme (Supplementary Fig. 6a ). We observed no overt histologic defects or perturbed distribution of antral epithelial proliferative or differentiation markers (Supplementary Fig. 6b ) and scRNA profiles of purified wild-type (WT) and Fgf7 −/− antral epithelium showed intact proportions and expression characteristics of proliferative and differentiated cells (Supplementary Fig. 6c ), with only subtle differences in foveolar cell transcripts between Fgf7 −/− and WT mice (Supplementary Data 3 ). Thus, despite the abundance and specificity of Fgf7 expression in a spatially discrete subpopulation of antral SEMFs and its budding effect in vitro, its essential, non-redundant role in maintaining antral epithelium in vivo is at most minor. Spatially and molecularly distinct corpus and antral PDGFRA Lo cell populations Next, we examined gastric Pdgfra + cell clusters other than Pdgfra Hi (Fig. 3 ). Considered separately from SEMFs, Pdgfra Lo and Pdgfra Int resolved into 5 sub-groups within 3 clusters; the smallest and most distinct cluster corresponds to CorpLo1 and few antral Pdgfra Lo cells, while the remaining cells cluster by corpus and antral origins (Fig. 5a ). Within the large corpus cluster, one sub-group, CorpLo2, shares expression of a panel of niche factor genes with AntLo, while the other sub-group, CorpLo3, expresses genes (e.g., Pappa , Sox11 , Postn , Nrg1 —see Fig. 3e ) that mark AntInt (Fig. 5a ). These populations selectively express BMPs, which inhibit ISCs, and non-canonical Wnts, which lack known niche function (Fig. 5a, b ). Conversely, factors known to constitute the ISC niche, such as Grem1 and Rspo3 , are selectively enriched in AntLo, CorpLo2, and the isolated corpus cluster CorpLo1 (Fig. 5a, b ). Thus, scRNA data separate gastric Pdgfra Lo cells into fractions that superficially resemble cells active in the ISC niche (AntLo, CorpLo1, CorpLo2) and those that express distinct, potentially opposing factors (AntInt and CorpLo3). Fig. 5: Identification and localization of Cd55 -expressing gastric PDGFRA Lo cells. a In isolation, gastric PDGFRA + mesenchyme other than SEMFs resolves into five subpopulations: previously identified AntInt, AntLo and CorpLo1 (Fig. 3 ) and two CorpLo subpopulations, CorpLo2 and CorpLo3. Relative expression of selected scRNA-seq markers is plotted below. Circle diameters: cell fraction expressing a gene, fill shades: normalized average expression. CorpLo3 shares markers identified in AntInt (see Fig. 3e ). b Bmp5, Bmp7, Wnt4, Grem1, Rspo3 , and Ctgf transcript densities projected on the UMAP plot of resolved non-SEMF cell clusters. CorpLo3 and AntInt express BMPs and Wnt4 , while AntLo, Corp1, and Corp2 express Grem1, Rspo3 , and Ctgf . Dashed lines mark the distinct populations. c Left: Relative Cd55 and Cd34 expression in sub-epithelial cell fractions from scRNA-seq analysis. Circle diameters and fill colors represent the parameters defined in ( a ). Middle: Relative Cd55 expression in PDGFRA Lo subpopulations. Right: Projection of Cd55 density on the PDGFRA Lo UMAP, showing nearly exclusive expression in CorpLo1, CorpLo2 and AntLo cells. d In situ hybridization (RNAscope) of corpus tissue sections, together with LAM immunostaining, localizes Cd55 in the epithelium (white arrows) and in PDGFRA Lo mesenchymal cells (orange arrows) near the gland base, on both sides of muscularis mucosae. The area within the dashed box is magnified below. Images represent scores of fields examined in two independent experiments. Scale bars 50 μm. e In situ hybridization (RNAscope) of corpus tissue sections localizes Grem1 (left) and Rspo3 (middle) near the gland base. Images represent scores of fields examined in two independent experiments. Scale bars 50 μm. Dotted lines mark the muscularis mucosae. In the heatmap, fluorescence signal strength is quantified along 50–52 individual glands. Source data are provided as a Source Data file. f In situ hybridization (RNAscope) of corpus tissue localizes Grem1 in the SMA1-immunostained muscularis mucosae, demarcated by dotted lines, and in the space corresponding to PDGFRA Lo cells near the gland base ( n = 2 independent experiments). Scale bars 50 μm. g Schematic illustration of the distribution of CD55 + PDGFRA Lo cells relative to corpus glands and the muscularis mucosae (MM). Grem1 - and Rspo3 -expressing cells lie largely beneath glands. Full size image To assess niche cell functions in isolated gastric cell populations, we sought a cell surface marker that could separate Pdgfra Lo cell fractions expressing Grem1 , Rspo3 or Ctgf (to varying degrees—shaded pink in Fig. 5a ) from those expressing BMP and non-canonical Wnts (shaded orange). In scRNA analysis, two cell surface marker genes, Cd34 and Cd55 , showed selective expression in AntLo, CorpLo2, and especially CorpLo1 cells (Fig. 5a ). Cd34 , a known marker of trophocytes and other intestinal PDGFRA Lo cells, is also abundant in endothelial cells [33] , [54] (Fig. 5c ). In contrast, Cd55 , which encodes the tetraspanin CD55 and marks SI mesenchymal cells that support in vitro expansion of SI crypts [35] , is additionally expressed only in a small fraction of gastric immune cells (at levels lower than in Pdgfra Lo cells—Fig. 5c ) and in the foveolar epithelium (Supplementary Fig. 7a ). Flow cytometry of epithelial (EpCAM + , Supplementary Fig. 7b ) and PDGFRA neg non-immune (CD45 − /PTPRC − ) cells from Pdgfra H2BeGFP mice showed negligible surface CD55 expression, but reliably purified corpus and antral CD55 + PDGFRA Lo cells (Supplementary Fig. 7c, d ) and traced CD55 expression in CD45 + /PTPRC + cells mostly to B lymphocytes (Supplementary Fig. 7e ). In fact, ~90% of B lymphocytes from each region expressed CD55 against 60% of myeloid cells and 70% of T lymphocytes. Whereas immunohistochemistry with multiple CD55 antibodies gave high background signals, in situ hybridization (ISH) with Cd55 probe showed that extra-epithelial Cd55 expression is restricted to sub-glandular mesenchymal cells located below and just above the muscularis mucosae, into the bottom ~1/6 of corpus gland height (Fig. 5d ). To better define this mesenchymal Cd55 + population, we used ISH probes for Grem1 and Rspo3 , which scRNA-seq detected in CorpLo1 or in CorpLo1 and CorpLo2, respectively (Fig. 5a —high Ctgf ISH signals in corpus SEMFs occluded Ctgf -expressing PDGFRA Lo cells). In Pdgfra H2BeGFP mouse corpus, Grem1 and Rspo3 localized in adjacent sub-glandular mesenchymal cell layers (Fig. 5e ). SMA1 (smooth muscle actin1, Fig. 5f ) immunostaining placed the dense ISH signals in a tissue layer where PDGFRA Lo cells intermingle with muscularis mucosae, while sparser signals localized to PDGFRA Lo cells located between the muscularis and the corpus gland base (Fig. 5f ). This distribution resembles that of Cd55 but the latter extends farther below the muscularis mucosae than Rspo3 and especially Grem1 (Fig. 5d–f ). Taken together with scRNA-seq, which showed broader expression of Cd55 than the other markers (Fig. 5a ), these findings indicate that CorpLo1 cells lie within and above the muscularis, CorpLo2 cells extend below the muscularis, and the largest subpopulation, CorpLo3 which lacks Grem1 or Rspo3 , surrounds the top and middle zones of corpus glands (Fig. 5g ). Extra-epithelial Cd55 in the antrum also localized in sub-glandular mesenchyme (Fig. 6a ). Consistent with low Rspo3 expression in scRNA-seq data (Fig. 5a ), ISH signals for Rspo3 were weak, but Grem1 and Ctgf localized confidently in sub-glandular mesenchyme, overlapping with Cd55 (Fig. 6b, c ): Grem1 + Pdgfra Lo cells are mixed with muscularis mucosae and Ctgf + Pdgfra Lo cells reside between the muscularis and antral gland bottoms. Thus, Cd55 + Pdgfra Lo cells are restricted to the space beneath both corpus and antral glands. ISH and scRNA-seq data were consistent in indicating that Rspo3 , when present, is co-expressed with Grem1 , but the overlap between Ctgf and Grem1 is limited in both stomach regions (Supplementary Fig. 8a ). The CD55 + fraction therefore represents a sub-glandular mix of Grem1 + Rspo3 + and Grem1 − Ctgf + cells. Fig. 6: Niche activity of gastric CD55 + PDGFRA Lo cells. Antral in situ hybridization localized ( a ) Cd55 to the epithelium (white arrows) and PDGFRA Lo mesenchymal cells (orange arrows) near gland bottoms; ( b ) Grem1 and Ctgf near the gland base (dotted lines demarcate glands, heatmaps: fluorescence along individual glands, n = 35 to n = 39, Source data provided as a Source Data file); and ( c ) Grem1 in SMA1 + muscularis mucosae, extending into sub-glandular PDGFRA Lo cells (dashed lines demarcate glands). Dashed boxes are magnified below ( a ) or to the right ( b , c ). Images represent fields examined in 2 ( a , c ) or 3 ( b ) independent experiments. Scale bars 50 μm. d Schema of mesenchymal cell distributions. MM muscularis mucosae. e Co-culture of gastric glands with CD55 + or CD55 − PDGFRA Lo cells from each region. ENRWG corpus n = 4, antral n = 12; CD55 + corpus n = 4, antral n = 11; CD55 − corpus n = 5, antral n = 9; No cells corpus n = 4, antral n = 11. Bars: mean ± SEM. Significance: one-way ANOVA and Tukey’s multiple comparison test. ns not significant. Source data provided as a Source Data file. Scale bars 400 μm. f Spheroid formation from SI crypts and antral or corpus glands co-cultured with CD55 + (gastric) or CD81 + (SI trophocyte) fractions from each region. SI crypts: CD81 + n = 6, Antral CD55 + n = 5, Corpus CD55 + n = 3; Antral glands: SI CD81 + n = 12, Antral CD55 + n = 11, Corpus CD55 + n = 3; Corpus glands: SI CD81 + n = 4, Antral CD55 + n = 3, Corpus CD55 + n = 4. n : independent experiments, each with ≥2 technical replicates. Bars: mean ± SEM. Significance: one-way ANOVA and Tukey’s multiple comparison test. ns not significant. Source data provided as a Source Data file. g Co-culture of gastric glands with or without corresponding CD55 + PDGFRA Lo cells, growth factors (+GF or −GF), and Porcupine inhibitor Wnt-C59 (Pi) or BMP2/4/7 cocktail (Bs). Bars: mean ± SEM. No cells+GF corpus n = 16, antral n = 24; −CD55 + +Pi corpus and antral n = 9, −CD55 + +Bs corpus n = 8, antral n = 7; −GF corpus n = 18, antral n = 25; +CD55 + corpus n = 13, antral n = 18; +CD55 + +Pi corpus n = 12, antral n = 8; +CD55 + +Bs corpus n = 13, antral n = 9. Significance: one-way ANOVA and Sidak’s multiple comparison test. ns not significant. Source data provided as a Source Data file. Scale bars 400 μm. Full size image These findings highlight similarities and differences between corpus, antral, and SI Pdgfra Lo mesenchyme. Antral Pdgfra Lo cells express less Grem1 or Rspo3 than their SI counterparts (Fig. 2g ), but the transcripts show substantively similar distribution in both sites, near proliferative and Lgr5 + stem cells at the base of antral glands and SI crypts (Fig. 6d ). The apparent gradient of high to low Grem1 and Rspo3 expression (from muscularis to epithelium) in sub-glandular corpus Pdgfra Lo cells also resembles a self-organized gradient recently described in the SI [35] (Fig. 5g ). However, proliferative and presumptive stem cells in the isthmus of corpus glands lie far from Grem1 - and Rspo3 -expressing cells. Therefore, sub-glandular CD55 + cells may drive isthmus cell replication from a distance, may act principally on nearby facultative stem cells in the gland base, or may affect epithelial differentiation more than cell replication per se. BMP signaling, for example, is implicated not only in exit from the stem-cell compartment [55] , [56] , [57] but also in intestinal endocrine [58] and gastric foveolar (pit) cell [25] differentiation. PDGFRA Lo cell populations that affect epithelial growth in vitro and differentiation in vivo Gastric mesenchymal PDGFRA Lo cells support gastric spheroid, but not intestinal organoid, growth in vitro (Fig. 2a, b ). To define the niche activities of the sub-glandular fraction, we used flow cytometry to isolate CD55 + and CD55 − cells from Pdgfra H2BeGFP mice (Supplementary Fig. 7b, c ), then co-cultured gastric glands with one cell fraction or the other in media lacking recombinant factors. While glands cultured with no mesenchymal cells or with CD55 − cells from antral or corpus mesenchyme generated at most a few tiny spheroids, those cultured with CD55 + cells robustly stimulated spheroid growth (Fig. 6e ). Like unfractionated gastric PDGFRA Lo cells (Fig. 2a ), neither fraction induced organoid formation from SI crypts, but both CD81 + SI trophocytes and CD55 + gastric PDGFRA Lo cells induced spheroid growth from isolated corpus and antral glands (Fig. 6f ). To define the signaling pathways most pertinent in the cellular effect of CD55 + cells, we added the Porcupine inhibitor Wnt-C59, which impairs secretion of all Wnts [59] , or a cocktail of recombinant BMPs 2, 4 and 7, to gastric gland co-cultures. While Wnt-C59 attenuated CD55 + cell effects on corpus and antral glands, BMP2/5/7 inhibition was significant on corpus, but statistically insignificant on antral glands (Fig. 6g ). Thus, only the CD55 + fraction of PDGFRA Lo cells can elicit gastric spheroids, owing in part to functions that BMPs and impaired Wnt secretion can override. Spheroid growth from gastric glands may reflect an experimental feature (close apposition of mesenchymal cells to epithelium) that differs from the native tissue structure, at least in the corpus where CD55 + PDGFRA Lo cells localize far from the isthmus. In the absence of a means to test the function of the full CD55 + cell fraction in vivo, Grem1 DTR mice [35] provided a path to deplete at least the minority Grem1 + subpopulation. Ablation of intestinal Grem1 + cells, including PDGFRA Lo CD81 + trophocytes, rapidly depletes overlying ISCs and progenitors [33] ; in line with this finding, treatment of Grem1 DTR mice with Diphtheria toxin resulted in >90% and ~50% depletion of Grem1 and Rspo3 transcripts (Fig. 7a ) and in arrested SI epithelial replication within attenuated crypts (Supplementary Fig. 8b ). In contrast, KI67 immunostaining revealed no compromise of corpus or antral epithelial proliferation (Fig. 7b ); the only consistent defect was near absence of antral UEAI staining (Fig. 7b ), signifying absent or defective basal mucous cells (see also Supplementary Fig. 1b ). Ablation of gastric Grem1 + cells elicited minor reductions in antral RNA levels of Lgr5 and the proliferative isthmus cell marker Stmn1 [14] , altered Muc6 levels in corpus and antrum, and reduced Troy mRNA in the corpus (Fig. 7b ). These findings identify selective and modest effects of Grem1 + cells on corpus and antral basal cell markers, implying that most of the CD55 + cell effect on gastric spheroids reflects Grem1 − ( Ctgf + ) cell activity. Fig. 7: Effects on gastric glands from ablation of Grem1 -expressing cells. a Grem1 DTR mice treated with Diphtheria toxin (DT) and untreated control mice were used to assess the effects of partial ( Grem1 + fraction) ablation of the CD55 + PDGFRA Lo cell compartment. Grem1 and Rspo3 mRNA levels were significantly reduced 72 h after DT treatment ( n = 4). Bars represent mean ± SEM values. Significance of differences was determined by two-tailed unpaired Student’s t test. * p < 0.05; ** p < 0.01; **** p < 0.0001. b Top: histology (H&E), KI67 immunofluorescence, and staining with fluorescent GSII and UEAI lectins to highlight proliferative and distinct mucous cell types in the corpus and antrum of DT-treated mice and untreated (No DT) controls. Scale bars 50 μm. Blue, DAPI; magenta, KI67; red, GSII; green, UEAI. Bottom: qRT-PCR analysis of corpus and antral epithelial cell markers (relative to Gapdh and to untreated controls, no DT) in tissues harvested 72 h after treatment ( n = 4). Bars represent mean ± SEM values. Significance of differences determined by two-tailed unpaired Student’s t test. Source data are provided as a Source Data file. c Schematic representation of all antral PDGFRA + cell types in relation to glandular epithelium. Full size image To ensure a proper epithelial census, microenvironments around specific zones in intestinal crypts and gastric glands generate Wnt, BMP, and other signaling gradients that balance cell self-renewal against differentiation [7] , [22] , [28] , [56] , [60] . Among mesenchymal cells, PDGFRA + cells as a group show the most regional diversity. In the intestine, they provide canonical Wnt ligands [35] and create the requisite BMP gradient [33] , but signaling sources and cellular arrangements are not known in the gastric corpus and antrum, where gland structures differ markedly [37] . Our bulk and single-cell RNA profiles, high-resolution microscopy, and gastric gland co-cultures identify spatially, molecularly, and functionally distinct PDGFRA + cell types. One large PDGFRA + cell type in the corpus and antrum expresses high Pdgfra and BMP and EGF ligand mRNAs, lies within basement membranes, and fails to induce spheroids in co-culture assays. In these respects, gastric Pdgfra Hi cells resemble intestinal SEMFs [33] , [61] , [62] , [63] , also called “telocytes” [31] , [64] . Pdgfra Hi cell aggregates surround antral gland pits, far from stem cells in gland bottoms and reminiscent of ISEMF density at crypt and villus tops [33] , [64] . Tight clustering of corpus Pdgfra Hi cells in nearest-neighbor space suggests that they are likely uniform along the gland length. In contrast, peri-foveolar antral SEMFs differ from corpus SEMFs and deep antral SEMFs in high expression of Fgf7 , Nrg1 , and other factors, but Fgf7 deletion alone had subtle effects on pit cell gene expression. Nevertheless, high and specific Fgf7 expression in peri-foveolar antral SEMFs and rFGF7 stimulation of budding in vitro suggest possible roles in non-homeostatic conditions. All other gastric PDGFRA + mesenchymal cells express lower levels of Pdgfra and BMP and EGF ligand mRNAs, lie farther from the epithelium than SEMFs, and elicit spheroid growth from gastric glands in the absence of supplemental growth factors. In both corpus and antrum, this in vitro trophic activity maps to CD55 + cells that reside beneath the gland base in vivo. Antral Cd55 expression and, by extension, in vitro trophic activity is limited to AntLo cells, distinct from Cd55 − AntInt. Furthermore, Cd55 expression is highly correlated with Ctgf , which localizes in the immediate vicinity of antral stem cells. These findings suggest a model wherein antral Pdgfra Lo cells segregate into a niche-active CD55 + fraction located near epithelial stem cells and inactive CD55 − AntInt. The minimal effects from ablation of Grem1 DTR cells in vivo imply that the stem cell support evident in vitro arises from the Grem1 − ( Ctgf + ) subpopulation of sub-glandular CD55 + cells. Nevertheless, anatomic and functional parallels with the sub-cryptal SI stem-cell niche are striking. Furthermore, the gene signature of corpus and antral CD55 + cells overlaps with that of colonic Fibroblasts 3a (“interstitial fibroblasts”) recently defined as a population lying below colonic crypts and expressing Cd55 and Grem1 among other genes [65] . The same gene signature also overlaps materially with the resting fibroblast population “F01” recently identified in human gastric cancer specimens [66] . Intestinal trophocytes are CD34 + CD81 + PDGFRA Lo cells that lie beneath the muscularis mucosae and robustly support spheroid formation from SI crypts; [33] , [36] however, supportive niche activity extends above the muscularis mucosae, into peri-cryptal CD81 − CD55 + PDGFRA Lo cells [35] . Thus, common features of antral and intestinal cells with demonstrable in vitro niche activity include PDGFRA (lower than in SEMFs) and CD55 expression, low levels of BMP ligand genes Bmp2/5/7 , and residence near stem cells. CD55 is a robust surface marker of these uniquely functional cells, in part supplanting CD81, which marks the most potent cells but is useful for cell isolation only from Pdgfra H2BeGFP mice (PDGFRA Ab only stains SEMFs reliably; most intestinal PDGFRA Lo cells escape Ab detection). We therefore propose to redefine “trophocytes” as the niche-active CD55 + mesenchymal cell fraction in both intestine and antrum. This definition has the practical advantage that CD55 + mesenchymal cells can be isolated by FACS from any mouse strain, not only from Pdgfra H2BeGFP , after straightforward exclusion of CD45 + lymphocytes and, for certainty, also EPCAM + epithelial cells ( Cd55 RNA is expressed in gastric epithelium, but flow cytometry did not detect the protein on cell surfaces). Notably, both corpus and antral CD55 + cells triggered spheroid formation from homologous or heterologous glands but not from SI crypts; this may be because Rspo3 and Grem1 , essential trophic factors for ISCs, are expressed at lower levels than in intestinal trophocytes. The functions of CD55 − PDGFRA Lo cell fractions, including AntInt and CorpLo3, remain unknown in any region of the digestive tract. CD55 expression is modulated by cytokines in other tissues [67] , [68] , [69] ; we investigated CD55 only as a molecular marker and did not ask whether its RNA and protein levels are similarly modulated in gastric epithelium, mesenchyme or lymphocytes. Constructing a parallel model for corpus Pdgfra Lo cells poses challenges, in part because a conceptual framework for the mesenchyme’s influence on active isthmus and facultative basal stem cells is still lacking. Pdgfra Lo cells in the corpus are more heterogeneous than those in the antrum, with CorpLo1 clustering far apart from CorpLo2 and CorpLo3 (Fig. 5a ), and Cd55 is expressed in both CorpLo1 and CorpLo2. As in the antrum, Cd55 -expressing Pdgfra Lo cells lie between the corpus gland base and muscularis mucosae, but unlike the antrum, this location is not near active isthmus stem cells. Therefore, the effect of corpus CD55 + cells in spheroid assays might represent their action on facultative stem cells or suggest that they influence isthmus stem cells from a distance in vivo; alternatively, it may reflect a fortuitous consequence of artificial epithelial-mesenchymal cell juxtaposition in spheroid assays. Recalling that Pdgfra Lo cells along the length of corpus glands lack Cd55 and are sparse near the isthmus (see Supplementary Fig. 1g ), another intriguing possibility is that isthmus stem cells derive their state from a combination of CD55 + cells acting from a distance and the paucity of CD55 − cells in their immediate vicinity. In summary, we report spatial, molecular, and functional features of gastric PDGFRA + mesenchyme at high resolution, noting salient differences between gastrointestinal regions (Fig. 7c ). Our findings identify CD55 as a robust surface marker of spatially segregated PDGFRA Lo cells with demonstrable niche activity in vitro, distinct from CD55 − cells that are inert in spheroid assays, and establish a foundation for further investigation of gastric mesenchymal niches in homeostasis and disease. Mouse models and treatment All animal procedures were approved by Animal Care and Use Committees at the Dana-Farber Cancer Institute or Columbia University Medical Center. Mice were housed in a pathogen-free animal facility and maintained on a 12-h light/dark cycle at constant temperature and humidity, with ad libitum access to food and water. Strains were maintained on a mixed C57BL/6 background. Male and females aged 8–16 weeks were used. Genotypes were identified by PCR analysis of genomic DNA isolated. Pdgfra H2BeGFP (JAX strain 007669), Pdgfra Cre(ER-T2) (JAX strain 032770), Rosa26 Lsl-TdTomato (JAX strain 007908), and Rosa26 mT/mG (JAX strain 07676) mouse strains were purchased from Jackson Laboratories. Grem1-P2A-DTR-P2A-TdTomato ( Grem1 DTR ) mice were described previously [35] . Rosa26 mT/mG mice were crossed with Pdgfra Cre(ER-T2) to generate compound heterozygotes. Cre recombinase activity was induced by intra-peritoneal (i.p.) injection of 2 mg tamoxifen (Sigma-Aldrich T5648) on 4 consecutive days, followed by visualization of Pdgfra -expressing cells. Fgf7 fl/fl mice, generated as described below, were crossed with Pdgfra Cre(ER-T2) and Rosa26 Lsl-TdTomato to obtain Pdgfra Cre(ER-T2) ;Fgf7 fl/fl ; Rosa26 LSL-TdTomato mice, and tamoxifen 2 mg/day was injected i.p. to induce cell-specific Cre activation and genetic recombination. Cre -negative littermates were used as controls. Grem1 DTR mice were treated with two i.p. injections of 50 μg/kg of Diphtheria toxin (DT, Sigma-Aldrich, D0564) on alternate days and harvested 24 h after the second injection. Fgf7 conditional mice A floxed conditional Fgf7 allele was generated by genome editing in 1-cell embryos. The targeting construct consisted of the Fgf7 exon 2 sequence flanked by LoxP sites and surrounded by short homology arms in an adeno-associated virus (AAV) vector. This vector was electroporated along with Cas9 protein and two sgRNA, as previously described [70] . Single-nucleotide substitutions at the PAM motifs were included in the targeting vector to prevent re-cutting after homologous recombination. 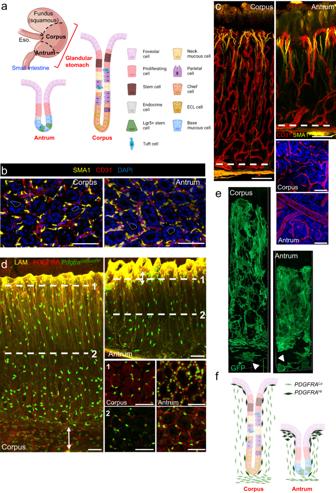Fig. 1: Structure and organization of gastric corpus and antral mesenchyme. aStomach and intestinal regions and different organizations of glandular stomach epithelia.bCross-sections of corpus (top) and antrum (bottom), showing smooth muscle actin (SMA1, yellow)-expressing smooth muscle fibers and CD31+(red) capillaries packed tightly in the stroma between glands (nuclei stained with DAPI, blue). Dashed lines delineate gland lumen. Scale bars 50 μm. Representative images from three independent experiments.cWhole-mount 3D rendering of corpus (left) and antral (right) glands, highlighting structural differences in muscle fibers (SMA1, yellow) and capillaries (CD31, red) in the two regions. Tissue cross-sections at the level marked by dashed lines are shown in the bottom right (DAPI in blue, CD31 in red). Scale bars 50 μm.dWhole-mount 3D rendering of corpus (left) and antral (top right) glands inPdgfraH2BeGFPmice. Laminin (yellow) marks the basal lamina and highlights gland pits. Tissue cross-sections at the levels marked 1 and 2 are shown in the bottom right, with PDGFRAHicells in neon green and PDGFRALocells in light green. Double-headed arrow highlights PDGFRALolayer beneath corpus gland bottoms. Immunostaining with PDGFRA antibody (red) shows the extent of PDGFRA+cytoplasm enveloping each gland. Scale bars 50 μm.eSingle frames extracted from 3D video renderings ofPdgfraCre(ER-T2);Rosa26mT/mGmouse (stained green after tamoxifen treatment) corpus (left) and antrum (right) to show the morphology ofPdgfraHicells enveloping each gland and additionalPdgfraLocells occupying space beneath glands (white arrowheads). Full videos of corpus and antral gland 3D renderings are included in the Supplementary information, see Supplementary Movies5and6.fSchematic representation of the distributions of PDGFRAHi(dark green) and PDGFRALo(light green) cells in relation to corpus and antral glands. Oligonucleotides used for in vitro transcription of sgRNAs and for genotyping are reported in Supplementary Table 1 . Gastrointestinal organoid/spheroid culture Organoids and spheroids were generated from wild-type mouse SI crypts or gastric glands. Crypts were isolated from the first half of the SI by incubating the tissue at 4 °C in cold 2 mM EDTA in phosphate-buffered saline (PBS), as described previously [42] . Crypts were plated in 5 μl Matrigel (Corning 356234) droplets and cultured in ENR medium: DMEM/F12 medium supplemented with 1X Glutamax, 10 mM HEPES, 1X penicillin/streptomycin, 1X normocin (Invivogen, ANT-NR-2), 1X primocin (Invivogen, ANT-PM-2), 1X N2 and B27 supplements (Life Technologies, 17502001 and 17504001), 1 mM N-acetylcysteine, 50 ng/ml murine rEGF (Peprotech, 315-09), 100 ng/ml murine rNOGGIN (Peprotech, 120-10C), and 10% Rspo1 conditioned medium (from 293T cells expressing mouse RSPO1). Glands were isolated from the gastric antrum or corpus by incubating the tissue in 10 mM EDTA in PBS at room temperature, as described previously [71] , [72] . Glands were separated from the stroma and muscularis by gentle scraping, washed in PBS, and cultured in ENR medium with addition of 10% Afamin/Wnt3a conditioned medium (MBL International, J2-001) and 10 nM gastrin (Sigma-Aldrich, G9145) or as specified in different experiments. Recombinant factors (human FGF10, Peprotech, 100-26; murine FGF7, Peprotech, 450-60; human BMP3, Peprotech, 120-24B; rat CTGF, R&D Systems, 92-37C-T050, Bmp2, Peprotech, 120-02C; murine BMP4, Peprotech, 315-27; human Bmp7, 120-03P) or Porcupine inhibitor Wnt-C59 (Thermo Fisher, NC0186427) were resuspended in 0.1% BSA in PBS and used at final concentrations of 100 ng/ml. Quantitation of mRNAs in gastric spheroids and in Grem1-DTR mouse tissues After 4 days of culture, Matrigel droplets were washed in cold PBS, detached gently from the plate, and incubated 20 min in cell recovery solution (Corning, 354270) to depolymerize the matrix. Spheroids were collected by centrifugation, resuspended in Trizol (Thermo Fisher Scientific), and total RNA was isolated with RNeasy Mini Kit (QIAGEN). One μg RNA was reverse transcribed using SuperScript III First-Strand Synthesis System (Invitrogen, 18080-051). Transcript levels were measured using Power SYBR Green (Life Technologies, 4367659) on a LightCycler 480 instrument (Roche) and normalized to Gapdh levels (2 −ΔCt ). Primer sequences are listed below. 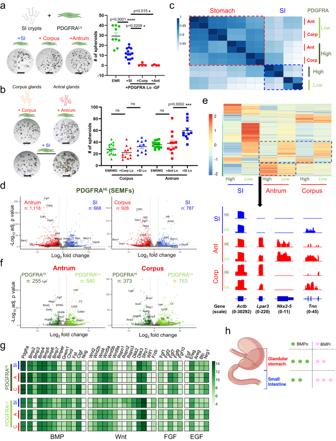Fig. 2: Molecular distinction of corpus and antral PDGFRA-expressing mesenchyme. aCo-culture of SI crypts with PDGFRALocells isolated from SI, antral or corpus mesenchyme and without NOG or RSPO1 (−GF). Stomach PDGFRALocells did not induce spheroids. SI organoid growth in complete ENR served as a control. Scale bars 400 μm. Bars represent mean ± SEM. ENR:n= 9, +SIn= 14, +Corp and +Ant:n= 4. Significance of differences determined by one-way ANOVA and Tukey’s multiple comparison test. ns not significant. Source data provided as a Source Data file.bCo-culture of corpus or antral glands with PDGFRALocells isolated from the same segment or from SI elicited spheroid growth in the absence of rNOG and RSPO1. Scale bars 400 μm. Corpus: ENRWGn= 15, +Corp Lon= 12, +SI Lon= 11, Antrum: ENRWGn= 14, +Ant Lon= 12, +SI Lon= 13. Control: gastric spheroid growth in ENRWG medium. Bars represent mean ± SEM. Significance of differences determined by one-way ANOVA and Sidak’s multiple comparison test. ns not significant. Source data provided as a Source Data file.cPearson correlations among RNA-seq libraries from SI, antral, and corpus PDGFRAHiand PDGFRALocells isolated fromPdgfraH2BeGFPmice. Differences between gastric and intestinal PDGFRA+cells are detailed in Supplementary Data1.dGenes differentially expressed (q< 0.05; log2fold-difference >1.5) between SI, antral, and corpus PDGFRAHicells. Selected genes are named. Significance of differences determined by DESeq2 default settings (Wald test).eGenes enriched in each regional population (q< 0.05; log2fold-difference >1.5;k-means = 6) and Integrative Genome Viewer tracks for representative genes enriched in antral PDGFRA+cells.Actbcontrols for normalization of read counts. Parentheses: range of signal values.fGenes differentially expressed (q< 0.05; log2fold-difference >1.5) between antral and corpus PDGFRAHiand PDGFRALocells. Significance of differences determined by DESeq2 default settings (Wald test).gRelative expression of mRNAs for candidate niche factors (BMP, Wnt, FGF, and EGF agonists and antagonists) in each mesenchymal cell population. Heatmap is prepared from normalized rlog counts from DEseq2; each row represents one replicate.hBulk RNA-seq data point to a higher BMP tone fromPdgfra+cells in stomach than in the SI. Similarly, corpus and antrum from Grem1 DTR mice treated with Diphtheria toxin and from untreated control animals were collected and processed for RNA isolation, cDNA synthesis, and quantitation of gene expression using primers reported in Supplementary Table 2 . Mesenchymal cell isolation SI, antral, and corpus mesenchyme was isolated as reported previously [33] , [38] , [54] . Tissue was harvested after perfusing adult Pdgfra H2BeGFP mice with cold PBS. After manual removal of external muscles, the epithelium was removed by rotating the tissue at 250 rpm in pre-warmed chelation buffer (10 mM EDTA, 5% fetal bovine serum (FBS), 1 mM Dithiothreitol, 10 mM HEPES in Hank’s Balanced Salt Solution, HBSS) for 20 min at 37 °C. The tissue was then washed with PBS and digested for 10 min at 37 °C in 3 mg/ml collagenase II (Worthington, LS004176) in HBSS supplemented with 5% FBS and 10 mM HEPES. Cells were harvested by centrifugation at 300 × g for 5 min For bulk RNA sequencing, cells were sorted on a BD FACSAria II cell sorter, gating on DAPI negative cells to identify live cells, and GFP to sort Pdgfra -high or -low expressing cells. Epithelial cell isolation To isolate epithelial cells, corpus and antrum were harvested from adult Pdgfra H2BeGFP mice perfused with cold PBS. Glands isolated as described above were digested first for 10 min at 37 °C in 3 mg/ml collagenase II (Worthington, LS004176) and 4X TrypLE (Thermo Fisher, A1217701) in DMEM supplemented with 1X penicillin/streptomycin on a rotating shaker, followed by incubation in 0.1 mg/ml DNase I (Worthington, LS002139) at 37 °C for an additional 5 min Enzymes were inactivated in DMEM + 10% FBS. Cells were collected by centrifugation (500 × g for 5 min), resuspended, and stained for FACS analysis. For scRNA-seq, cells were sorted on a BD FACSAria II cell sorter, gating on DAPI negative cells to identify live cells. For CD55 expression experiment, cells were stained with APC-conjugated EpCAM antibody (BioLegend, 118214, 1:100) and PE-conjugated CD55 antibody (BioLegend, 131803, 1:75). Gland and crypt co-cultures with mesenchymal cells Whole mesenchyme was isolated and plated on tissue culture plates (SI) or fibronectin-coated tissue culture plates (gastric mesenchyme, Corning, 354451) in DMEM/F12 medium supplemented with 10% FBS, 1X penicillin/streptomycin, 1X normocin, 1X primocin, 1X Glutamax, and 10 mM HEPES. Three days later, cells were washed in PBS, removed from the plates with 0.25% Trypsin (5 min at 37 °C), washed, and stained with antibodies. SI mesenchyme was stained with biotin-CD81 antibody (eBioscience, 13081181, 1:100) followed by incubation with streptavidin-APC-conjugated secondary antibody (eBioscience, 17431782, 1:100). Gastric cells were incubated with PE-conjugated CD55 antibody (BioLegend, 131803, 1:75) or, to isolate endothelial cells, with PE-conjugated CD31 antibody (BD Biosciences, 553373) and PE-Cy7-conjugated CD45 antibody (Invitrogen, 25-0451-82). FACS gating strategies are reported in Supplementary Fig. 9a . In total, 5000 viable FACS-sorted cells were co-cultured with ~20 glands or crypts in 5 μl Matrigel droplets in basal media (DMEM/F12 supplemented with 1X Glutamax, 10 mM HEPES, 1X penicillin/streptomycin, 1X normocin, 1X primocin, 1X N2 and B27 supplements, and 1 mM N-acetylcysteine) with no recombinant factors or as specified. Immunohistochemistry and FACS analysis Immunohistochemistry was performed on 10 μm fixed tissue sections prepared using a Leica cryostat on tissues frozen in OCT compound (Tissue-Tek, VWR Scientific, 4583). Whole-mount immunohistochemistry was performed as described [73] . Mice were perfused with ice cold PBS, followed by 4% paraformaldehyde (PFA). Antrum or corpus was pinned on agarose plates, treated with mucolytic solution (20 mM N-acetyl cysteine and 20 mM DTT in PBS) for 15 min at room temperature, and fixed for 15 min in 4% PFA. External muscle was removed manually before overnight fixation with 15% picric acid, 0.5% PFA in PBS. On day 2, tissues were washed in PBS and placed in 10% sucrose for 4 h, then 20% sucrose overnight at 4 °C. On day 3, tissues were placed in blocking buffer (0.5% bovine serum albumin, 0.6% Triton X-100, 0.05% goat serum, 0.0005% sodium azide) for 6 h, followed by overnight incubation with primary antibodies at 4 °C. On day 4, after 5 hourly washes in wash buffer (0.3% Triton X-100 in PBS), tissues were incubated at 4 °C with Alexa Fluor-conjugated secondary antibodies (Invitrogen) and DAPI (1:1000 dilution). The next day tissues were washed for 5 h with buffer changes every 30 min and fixed in 4% PFA at 4 °C for 1–2 days. Hand-cut 1 mm fragments were positioned on glass slides with imaging spacers (Grace Bio-Labs SecureSeal, Sigma-Aldrich), cleared for 30 min with FocusClear (CelExplorer, FC-101) at room temperature, and mounted with VectaShield (Thermo Fisher Scientific) medium. Tissues from at least three independent mice were imaged using an SP5X laser scanning confocal microscope (Leica Microsystems CMS GmbH) or an LSM980 microscope and ZEN Desk 3.4 software (Carl Zeiss GmbH). Images were analyzed using Fiji [74] and videos were generated with ZEN Desk 3.4 software. The following primary antibodies were used at 1:500 dilution unless otherwise specified: CD31 (BD Biosciences, 557355); Laminin (Sigma-Aldrich, L9393); alpha-smooth muscle actin1 (SMA1, Abcam, ab5694); PDGFRA (R&D Systems, AF1062, 1:100); MUC5AC (Cell Signaling Technology, 6119S); Gastrin (Abcam, ab232775, 1:100); and Somatostatin (Santa Cruz Biotechnology, sc-55565, 1:100). Alexa fluor 647-conjugated lectin GS-II (1:500, Life Technologies, L32451) and FITC-conjugated lectin UEAI (1:500, Life Technologies, L32476) were used to identify gastric mucous cell types. CD55 expression was analyzed on freshly isolated mesenchymal cells. Whole mesenchyme was isolated as described above. Cells were blocked for 15 min on ice with TruStain FcX PLUS (BioLegend, 156603) and stained for 20 min at room temperature with the following antibodies: BV711 anti-CD11b (BD Biosciences, 563168), Alexa Fluor 647 anti-CD19 (BioLegend, 115525), PE/Cy7 anti-CD3 (BioLegend, 100219), APC/Cy7 anti-CD45 (BioLegend, 103115), PE anti CD55 (BioLegend, 131803). After two washes, cells were incubated with DAPI (BD Biosciences, 564907) and analyzed with a BD LSR Fortessa cell analyzer. The gating strategy is reported in Supplementary Fig. 9 . RNA sequencing For bulk RNA sequencing, Pdgfra -expressing cells were isolated, FACS-sorted from antrum and corpus as described above, and placed in Trizol Reagent (Thermo Fisher Scientific). Total RNA was isolated with RNeasy Micro Kit (QIAGEN) and used for library preparation (5–10 ng) using SMART-Seq v4 Ultra Low Input RNA Kit (Clontech). For single-cell RNA sequencing, whole mesenchyme was isolated as described above and dead cells were eliminated by flow cytometry with DAPI stain. About 10,000 cells were loaded onto a 10X Genomics Chip G. Libraries were prepared according to the manufacturer’s protocol using Single-Cell 3’ v3.1 chemistry (10X Genomics, PN-1000128) and Libraries were sequenced on the Novaseq platform (Illumina). RNAscope in situ hybridization mRNA detection for spatial localization of cell populations was carried out using the RNAscope Multiplex Fluorescent Reagent Kit v2 (Advanced Cell Diagnostics) [33] , [75] . and probes designed by Advanced Cell Diagnostics: Cd55 (421251), Grem1 (314741), Ctgf (314541), Fgf7 (443521), Bmp3 (428461), Nrg1 (468841), and Rspo3 (483781). We followed the manufacturer’s recommended procedure, including 3 min (corpus) or 5 min (antrum) of target retrieval. As the procedure extinguished native GFP fluorescence, GFP signals were revealed by immunohistochemistry using GFP antibody (Abcam, ab6556, 1:100) as described previously [33] . Smooth muscle actin (SMA1, Abcam, ab5694) and Laminin (Sigma-Aldrich, L9393) antibodies were also used (1:100). Tissues were imaged using an SP5X laser scanning confocal microscope (Leica Microsystems CMS GmbH) or an LSM980 microscope and ZEN Desk 3.4 software (Carl Zeiss GmbH). Fluorescent signals along gastric glands were quantified with Fiji software. Data processing and analysis Image segmentation and quantitation GFP + cells were quantified using Cellpose plugin in CellProfiler [76] , [77] . Eight images were quantified per gastric region and representative examples are reported. Masks were generated using Cellpose pre-trained model “cyto2” and a cell diameter of 43 pixels. Each image contained about 300 segmented GFP + cells and >99% of cells were included in the segmentation. Segmented masks and original images were then fed into CellProfiler to quantify the distribution of GFP + cells. Signal intensity cut-offs to distinguish GFP Hi from GFP Lo cells were established from analysis of multiple cells. Data were represented graphically using Prism9 (GraphPad Inc). 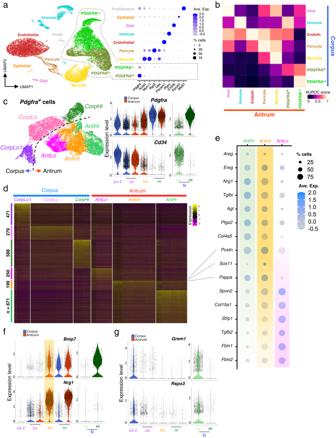Fig. 3: Delineation of corpus and antral PDGFRA+mesenchymal cell populations. aLeft: Uniform manifold approximation and projection (UMAP) plot of mRNA profiles from 34,445 single cells isolated from corpus (20,624 cells) and antral (13,821 cells) mesenchyme. Right: Relative expression of known cell-restricted genes in the UMAP cell clusters. Circle diameters represent the cell fraction expressing a gene and shades of purple represent normalized average expression within the population.bMetaNeighbour AUROC (area under the receiver operating characteristic) analysis shows high similarity between corresponding antral and corpus mesenchymal cells of each type other than the PDGFRAHiand PDGFRALocell populations.cLeft: UMAP identification of distinct populations ofPdgfra-expressing cells extracted from scRNA analysis of unfractionated mesenchyme. Right: Relative expression ofPdgfraandCd34in the identifiedPdgfra-expressing populations and the corresponding SI cells. Blue, corpus; red, antrum; green, SI. The 3 corpus populations are more distinct than the 3 antral populations.dDifferential genes expressed among the six PDGFRA+mesenchymal cell types (Wilcoxon Rank Sum test, logfc.treshold = 0.25). The genes are listed in Supplementary Data2.eRelative expression of marker genes from the three antral PDGFRA+subpopulations identified by scRNA-seq. Circle sizes represent the percentage of cells expressing a gene, fill colors represent normalized average expression. AntInt shows distinct intermediate patterns.fExpression of niche genesBmp7andNrg1in each population compared withPdgfra-expressing SI mesenchymal cells. AntInt expression levels are comparable to those in antralPdgfraHicells (AntHi).Nrg1expression in corpus and SI is significantly lower than in antral cells.gGrem1andRspo3expression in each population compared withPdgfra-expressing SI cells. Both genes are restricted toPdgfraLopopulations and expressed at lower levels in the stomach than in SI. Bulk RNA-sequencing Data were aligned to mouse reference genome mm10 using the Viper pipeline with default settings [78] and the quality was verified using RSeQC [79] . The R platform 4.2.1 was used for further analyses. Reads from genes known to express in gastric epithelium and genes encoded on sex chromosomes were excluded. Data were normalized and differential gene expression ( p adj < 0.05; |log 2 fold-change| > 1.5) was determined with the DESeq2 package [80] . Reads per kb per million tags (RPKM) values were generated from normalized counts. Pearson correlation coefficients were calculated from DESeq2 normalized counts and plotted using Corrplot package [81] . Principal component analysis (PCA) was done and heatmaps of selected genes were generated using Rlog-transformed counts. Integrative Genome Viewer (IGV) data tracks were generated from RPKM-normalized bigwigs loaded into IGV 2.15.4 (Broad Institute). Data from SI mesenchyme (GSE130681) were reported previously [33] . Single-cell RNA sequencing (scRNA-seq) Samples were aligned to the mm10 genome using 10x Genomics Cell Ranger 3.0.2 with default parameters [82] . Bioinformatic analyses were conducted using R version 4.2.1. Single-cell analyses used Seurat 4.1.0 [83] . Cells were filtered for <12% mitochondrial and >1000 unique reads. Data were merged and normalized using sctransform [84] . 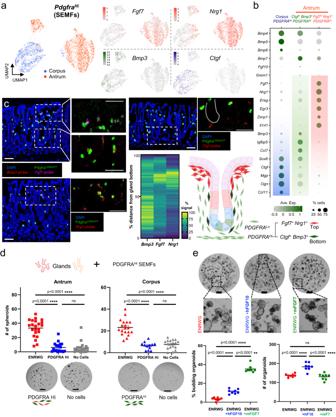Fig. 4: Identification and functional assessment of distinct gastric SEMF populations. aIn isolation, corpus and antral SEMFs are distinct and antral SEMFs divide further into two cell populations. Right:Fgf7,Nrg1,Bmp3, andCtgfmRNA densities projected on the UMAP plot.bRelative expression of scRNA-seq markers from the three SEMF populations. Circle diameters and fill colors represent the fraction of cells expressing a gene and normalized average expression levels. The two antral SEMF populations differ in expression ofFgf7, Nrg1,Bmp3, and other factors; corpus SEMFs resemble the smaller antralBmp3+cluster more than the larger population of antralFgf7+Nrg1+cells.cFluorescence in situ hybridization (RNAscope) on antral tissue sections localizesFgf7- andNrg1-expressing PDGFRAHiSEMFs near gland pits andBmp3- andCtgf-expressing cells in the lower half of glands. Images represent fields examined in three independent experiments with each probe. Scale bars 50 μm. Heatmap: average fluorescence signal quantified along 16–25 individual glands (Ctgfprobe quantification is shown in Fig.6a). Source data are provided as a Source Data file. Right: schematic representation of antral SEMF distribution.dCo-culture of antral and corpus glands with unfractionated PDGFRAHicells, which fail to induce spheroids in the absence of rNOG and RSPO1. Glands cultured in ENRWG medium serve as controls. Scale bars 400 μm. Bars represent mean ± SEM. Antrum: +ENRWGn= 22, +PDGFRAHin= 19, No cellsn= 22; Corpus: +ENRWGn= 19, +PDGFRAHin= 12, No cellsn= 18.n: number of culture wells analyzed over six independent experiments. Significance of differences determined by one-way ANOVA coupled with Sidak’s multiple comparison test. ****p< 0.0001, ns not significant. Source data are provided as a Source Data file.eAntral glands exposed to recombinant rFGF7 or rFGF10 in addition to complete ENRWG medium. Budding of spheroid structures increased upon treatment with rFGF7 without affecting spheroid numbers (n= 8 independent experiments). Bars represent mean ± SEM. Significance of differences determined by one-way ANOVA coupled with Dunnett’s multiple comparison test. ns not significant. Scale bars 400 μm. Source data are provided as a Source Data file. Cell features were detected with the FindVariableFeatures function (2000 features, selection method “vst ” ). The first 15 principal components were taken to run uniform manifold approximation and projection (UMAP) algorithms [85] . Cell types were identified using established marker genes detected by the “FindAllMarkers” function in Seurat2 (min.pct = 0.25, test “roc”). To assess similarities between gastric mesenchymal cell types, we used MetaNeighbor-AUROC analysis. Highly variable genes in the datasets were used to train an algorithm to predict the type of a given cell by the genes expressed in its nearest neighbors. To calculate similarity between cell types A and B across any pair of samples, the cell type annotation from one group was hidden and a score was used to represent how often a cell of type A is predicted to overlap with cells of type B vs. all other cell types (area under the receiver operating characteristic, AUROC score). Higher scores indicate greater similarity between two cell types. To address concerns about separation of Pdgfra + populations, we used AUGUR analysis [49] , which uses a regularized random forest classifier to directly quantify transcriptional differences between cell types under different conditions. High AUC scores indicate larger transcriptional difference between a given cell type in condition A vs. condition B (in this case corpus vs. antrum). Previously published scRNA-seq data from corpus epithelium were analyzed to determine Cd55 expression [14] , [21] , [86] . Cells were filtered for >200 unique reads and mitochondrial content <40%. Data were integrated based on a set of anchors between Seurat objects found using FindIntegrationAnchors, normalized using sctransform and analyzed as explained above. Statistics Prism9 (GraphPad Inc) was used for statistical analysis of all data. Specific tests and significance levels are indicated in figure legends. 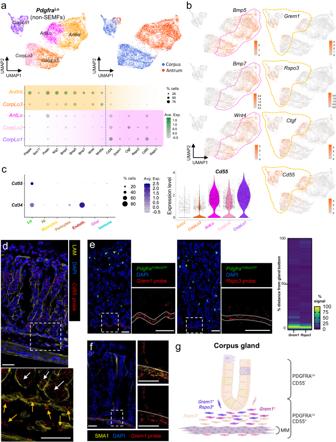Fig. 5: Identification and localization ofCd55-expressing gastric PDGFRALocells. aIn isolation, gastric PDGFRA+mesenchyme other than SEMFs resolves into five subpopulations: previously identified AntInt, AntLo and CorpLo1 (Fig.3) and two CorpLo subpopulations, CorpLo2 and CorpLo3. Relative expression of selected scRNA-seq markers is plotted below. Circle diameters: cell fraction expressing a gene, fill shades: normalized average expression. CorpLo3 shares markers identified in AntInt (see Fig.3e).bBmp5, Bmp7, Wnt4, Grem1, Rspo3, andCtgftranscript densities projected on the UMAP plot of resolved non-SEMF cell clusters. CorpLo3 and AntInt express BMPs andWnt4, while AntLo, Corp1, and Corp2 expressGrem1, Rspo3, andCtgf. Dashed lines mark the distinct populations.cLeft: RelativeCd55andCd34expression in sub-epithelial cell fractions from scRNA-seq analysis. Circle diameters and fill colors represent the parameters defined in (a). Middle: RelativeCd55expression in PDGFRALosubpopulations. Right: Projection ofCd55density on the PDGFRALoUMAP, showing nearly exclusive expression in CorpLo1, CorpLo2 and AntLo cells.dIn situ hybridization (RNAscope) of corpus tissue sections, together with LAM immunostaining, localizesCd55in the epithelium (white arrows) and in PDGFRALomesenchymal cells (orange arrows) near the gland base, on both sides of muscularis mucosae. The area within the dashed box is magnified below. Images represent scores of fields examined in two independent experiments. Scale bars 50 μm.eIn situ hybridization (RNAscope) of corpus tissue sections localizesGrem1(left) andRspo3(middle) near the gland base. Images represent scores of fields examined in two independent experiments. Scale bars 50 μm. Dotted lines mark the muscularis mucosae. In the heatmap, fluorescence signal strength is quantified along 50–52 individual glands. Source data are provided as a Source Data file.fIn situ hybridization (RNAscope) of corpus tissue localizesGrem1in the SMA1-immunostained muscularis mucosae, demarcated by dotted lines, and in the space corresponding to PDGFRALocells near the gland base (n= 2 independent experiments). Scale bars 50 μm.gSchematic illustration of the distribution of CD55+PDGFRALo cellsrelative to corpus glands and the muscularis mucosae (MM).Grem1- andRspo3-expressing cells lie largely beneath glands. Graphical drawings were created at BioRender.com. 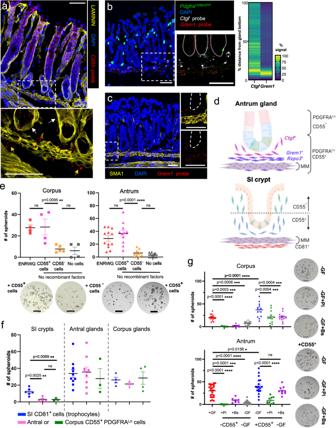Fig. 6: Niche activity of gastric CD55+PDGFRALocells. Antral in situ hybridization localized (a)Cd55to the epithelium (white arrows) and PDGFRALomesenchymal cells (orange arrows) near gland bottoms; (b)Grem1andCtgfnear the gland base (dotted lines demarcate glands, heatmaps: fluorescence along individual glands,n= 35 ton= 39, Source data provided as a Source Data file); and (c)Grem1in SMA1+muscularis mucosae, extending into sub-glandular PDGFRALocells (dashed lines demarcate glands). Dashed boxes are magnified below (a) or to the right (b,c). Images represent fields examined in 2 (a,c) or 3 (b) independent experiments. Scale bars 50 μm.dSchema of mesenchymal cell distributions. MM muscularis mucosae.eCo-culture of gastric glands with CD55+or CD55−PDGFRALocells from each region. ENRWG corpusn= 4, antraln= 12; CD55+corpusn= 4, antraln= 11; CD55−corpusn= 5, antraln= 9; No cells corpusn= 4, antraln= 11. Bars: mean ± SEM. Significance: one-way ANOVA and Tukey’s multiple comparison test. ns not significant. Source data provided as a Source Data file. Scale bars 400 μm.fSpheroid formation from SI crypts and antral or corpus glands co-cultured with CD55+(gastric) or CD81+(SI trophocyte) fractions from each region. SI crypts: CD81+n= 6, Antral CD55+n= 5, Corpus CD55+n= 3; Antral glands: SI CD81+n= 12, Antral CD55+n= 11, Corpus CD55+n= 3; Corpus glands: SI CD81+n= 4, Antral CD55+n= 3, Corpus CD55+n= 4.n: independent experiments, each with ≥2 technical replicates. Bars: mean ± SEM. Significance: one-way ANOVA and Tukey’s multiple comparison test. ns not significant. Source data provided as a Source Data file.gCo-culture of gastric glands with or without corresponding CD55+PDGFRALocells, growth factors (+GF or −GF), and Porcupine inhibitor Wnt-C59 (Pi) or BMP2/4/7 cocktail (Bs). Bars: mean ± SEM. No cells+GF corpusn= 16, antraln= 24; −CD55++Pi corpus and antraln= 9, −CD55++Bs corpusn= 8, antraln= 7; −GF corpusn= 18, antraln= 25; +CD55+corpusn= 13, antraln= 18; +CD55++Pi corpusn= 12, antraln= 8; +CD55++Bs corpusn= 13, antraln= 9. Significance: one-way ANOVA and Sidak’s multiple comparison test. ns not significant. Source data provided as a Source Data file. Scale bars 400 μm. 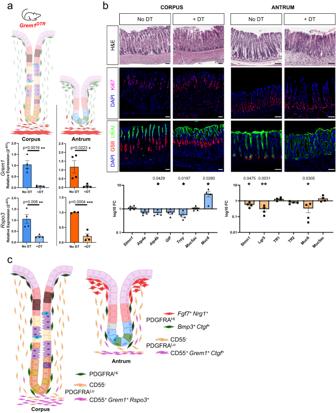Fig. 7: Effects on gastric glands from ablation ofGrem1-expressing cells. aGrem1DTRmice treated with Diphtheria toxin (DT) and untreated control mice were used to assess the effects of partial (Grem1+fraction) ablation of the CD55+PDGFRALocell compartment.Grem1andRspo3mRNA levels were significantly reduced 72 h after DT treatment (n= 4). Bars represent mean ± SEM values. Significance of differences was determined by two-tailed unpaired Student’sttest. *p< 0.05; **p< 0.01; ****p< 0.0001.bTop: histology (H&E), KI67 immunofluorescence, and staining with fluorescent GSII and UEAI lectins to highlight proliferative and distinct mucous cell types in the corpus and antrum of DT-treated mice and untreated (No DT) controls. Scale bars 50 μm. Blue, DAPI; magenta, KI67; red, GSII; green, UEAI. Bottom: qRT-PCR analysis of corpus and antral epithelial cell markers (relative toGapdhand to untreated controls, no DT) in tissues harvested 72 h after treatment (n= 4). Bars represent mean ± SEM values. Significance of differences determined by two-tailed unpaired Student’sttest. Source data are provided as a Source Data file.cSchematic representation of all antral PDGFRA+cell types in relation to glandular epithelium. No statistical method was used to predetermine sample size. No data were excluded from the analyses. The experiments were not randomized, and the investigators were not blinded to allocation during experiments and outcome assessment. Imaging experiments were repeated a minimum of three times with comparable results and representative images are reported in the study. Reporting summary Further information on research design is available in the Nature Portfolio Reporting Summary linked to this article.